Integration of molecular and enzymatic catalysts on graphene for biomimetic generation of antithrombotic species The integration of multiple synergistic catalytic systems can enable the creation of biocompatible enzymatic mimics for cascading reactions under physiologically relevant conditions. Here we report the design of a graphene–haemin–glucose oxidase conjugate as a tandem catalyst, in which graphene functions as a unique support to integrate molecular catalyst haemin and enzymatic catalyst glucose oxidase for biomimetic generation of antithrombotic species. Monomeric haemin can be conjugated with graphene through π–π interactions to function as an effective catalyst for the oxidation of endogenous L -arginine by hydrogen peroxide. Furthermore, glucose oxidase can be covalently linked onto graphene for local generation of hydrogen peroxide through the oxidation of blood glucose. Thus, the integrated graphene–haemin–glucose oxidase catalysts can readily enable the continuous generation of nitroxyl, an antithrombotic species, from physiologically abundant glucose and L -arginine. Finally, we demonstrate that the conjugates can be embedded within polyurethane to create a long-lasting antithrombotic coating for blood-contacting biomedical devices. Biological systems can often drive complex chemical transformations under mild conditions (for example, aqueous solution, physiological pH, room temperature and atmospheric pressure), which is difficult to achieve in conventional chemical reactions. This unique ability is generally empowered by a series of synergistic protein catalysts that can facilitate reaction cascades through complex metabolic pathways. There is significant interest in exploring molecular assemblies and/or conjugated catalytic systems as analogues to the functional proteins that can facilitate chemical transformations under biologically mild conditions [1] . Although ‘artificial enzymes’ have been studied for decades [2] , catalysts mimicking true enzymes for designated and complex reaction pathway have been much less frequently explored. The integration of enzymatic catalysts with molecular catalysts could create functional tandem catalytic systems for important chemical transformations not otherwise readily possible [3] , [4] . Despite the significant interest [5] , [6] , [7] , it is quite challenging to build a system that can allow enzymatic catalysts and molecular catalysts to operate synergistically under the same conditions (for example, aqueous solutions and physiological pH). Conjugation of these two distinct catalyst systems on a common platform support offers a plausible pathway. In this regard, the single-atom layer thick material graphene represents an interesting support for both enzymatic and molecular catalysts owing to several of its unique characteristics. First, bulk quantities of graphene flakes can now be readily prepared through chemical exfoliation of graphite oxide (GO) followed by chemical reduction [8] , [9] , [10] , [11] , [12] , [13] . Chemically reduced graphene typically possesses a large number of functional groups at the edges or defect sites to enable solubility/dispersibility in various solvents. These functional groups can also allow flexible covalent chemistry for linkage with molecular systems or enzymes. In addition, the extended π surface of graphene can also enable further functionalization via cation–π or π–π interactions. This rich surface chemistry offers excellent potential for coupling multiple distinct catalysts on graphene to create tandem catalysts for reaction cascading. Furthermore, the two-dimensional structure of graphene provides a unique geometry as a catalyst support with a large open surface area that is readily accessible to substrates/products with minimal diffusion barriers. Finally, it has been shown that graphene has better biocompatibility than other carbon nanomaterials for potential biomedical applications [14] . Thrombus formation is one of the most common and severe problems that lead to complications of blood-contacting biomedical devices including catheters, vascular grafts and heart valves [15] . Therefore, it is of considerable interest to develop an antithrombotic coating on biomedical devices that can sustain their functionality, decrease failure rate, and therefore greatly reduce associated medical complications and cost. Nitric oxide (NO) is recognized as a potent antiplatelet agent that can help prevent thrombus formation [16] . The extraordinary thrombo-resistant nature of healthy blood vessels is largely attributed to the continuous production of low fluxes ( ca. 0.5~4.0 × 10 −10 mol cm −2 min −1 ) of NO by the endothelial cells that line the inner walls of all blood vessels [17] . The design and fabrication of polymeric coatings capable of releasing or generating NO has recently drawn considerable attention for mitigating the risk of thrombus formation. A significant portion of the studies have focused on exogenous NO donors such as diazeniumdiolates [18] , which can immediately release NO when exposed to water or physiological environments (that is, blood, body fluids and so on). Such artificial polymeric coatings with embedded or covalently linked NO donors release NO to minimize thrombus formation [19] , [20] , [21] . However, the application of this approach for long-term implants, such as vascular grafts or haemodialysis catheters, is limited by the inevitable depletion of the finite reservoir of reagents in an exogenous NO donor source [22] . In addition, the labile nature of most NO donors (heat, light and moisture sensitivity) curtails their practical manufacturability and clinical applications. Moreover, the toxicity of some diazeniumdiolate precursors and the potential formation of carcinogenic nitrosamine by-products may also pose an adverse effect [23] . Alternatively, a surface coating capable of catalytic generation of NO from physiological components may offer a more attractive strategy for sustained NO release. For example, organoselenium [24] , [25] has been shown to trigger the decomposition of S -nitrosothiols, well-known endogenous NO carriers, to generate NO; this strategy is potentially useful for the continuous release of NO over long time periods. However, the relatively low level and highly variable concentrations of endogenous nitrosothiols in blood [26] limit the reliability of these NO-generating materials. In vivo toxicity studies also suggested that the reaction between reduced selenium species and oxygen is fast enough to produce a significant amount of superoxide that can react with NO to produce peroxynitrite, a toxic species [27] . In addition, selenium radical formation is also problematic, although aromatic organoselenium species have been found to be far less toxic (for example, ebselen [28] ). Biologically, NO is believed to arise from the oxidation of L -arginine catalysed by a family of nitric oxide synthase enzymes that utilize the reduced form of nicotinamide adenine dinucleotide phosphate (NADPH) as a cofactor along with O 2 as the oxidant [29] , [30] . Under conditions where the L -arginine concentration and/or cofactor supplies are limited, nitroxyl (HNO), the one electron reduced form of NO, can also be produced [31] . HNO has been studied extensively with regard to its provocative and pharmacological importance for heart failure treatment [31] , and it has recently been reported that HNO possesses antithrombotic activity analogous to NO [32] . Previous studies also indicate that hydrogen peroxide can substitute for NADPH and O 2 as the oxidant for HNO production [33] , [34] . Thus, biomimetic generation of antithrombotic HNO is a possible solution to the problems associated with NO-releasing materials and NO-generating catalysts. However, to date, there is no report of a biocompatible surface capable of local generation of HNO for effectively minimizing thrombus formation. Here we report a new design of graphene–haemin–glucose oxidase (GOx) conjugate as a tandem catalyst to enable the continuous generation of HNO from physiologically abundant glucose and L -arginine, and demonstrate that the integrated tandem catalyst can be used to create a long-lasting antithrombotic coating. The design of graphene–haemin–GOx tandem catalyst Haemin, an iron porphyrin species, is the catalytic centre of nitric oxide synthase. Free haemin itself is generally inactive as a catalyst because it undergoes molecular aggregation and oxidative destruction under physiological conditions [35] . Resin-supported hydrophilic iron porphyrin derivatives have previously been shown to be active for the oxidation of L -arginine, but with a rather limited turnover number due to a rapid loss of catalytic activity [36] . This system is also not suitable for practical clinical applications because it requires a high concentration of H 2 O 2 oxidant (38 mM), well beyond the physiological concentration. Recent studies have shown that monomeric haemin can be immobilized onto graphene to form a stable graphene–haemin conjugate that exhibits peroxidase-like activity for a variety of biomimetic oxidation reactions, using H 2 O 2 as the oxidant [37] , [38] . To create the tandem catalyst, we immobilized monomeric haemin onto graphene through π–π interactions and covalently linked GOx with graphene to form a graphene–haemin–GOx conjugate ( Fig. 1 ). With the integration of GOx in the conjugates, we expect to produce H 2 O 2 locally from endogenous glucose for the subsequent haemin-catalysed oxidation of L -arginine to generate antithrombotic HNO species. In this way, this complex conjugate can be used as an effective biomimetic catalyst for the generation of HNO species using only endogenous species, namely, glucose and L -arginine. Importantly, the physiological concentrations of glucose, L -arginine and the required HNO levels for antiplatelet activity follow a nearly ideal cascade: blood glucose concentration is ca. 2–5 mM, capable of creating more than enough peroxide to oxidize L -arginine, which is present at ca. 200 μM. The amount of HNO necessary for significant antithrombotic effects is probably in the sub-μM range [32] , which is at least three to four orders of magnitude lower than actual L -arginine concentrations. 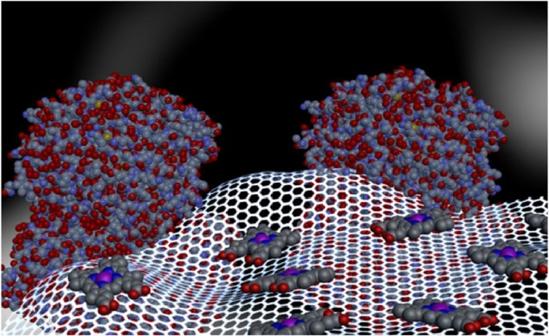Figure 1: Schematic illustration of graphene–haemin–GOx conjugates. Monomeric haemin molecules are conjugated with graphene through π–π interactions to function as an effective catalyst for the oxidation ofL-arginine, and GOx is covalently linked to graphene for oxidation of glucose and local generation of H2O2. Figure 1: Schematic illustration of graphene–haemin–GOx conjugates. Monomeric haemin molecules are conjugated with graphene through π–π interactions to function as an effective catalyst for the oxidation of L -arginine, and GOx is covalently linked to graphene for oxidation of glucose and local generation of H 2 O 2 . Full size image Graphene–haemin for HNO production The catalytic oxidation characteristics of graphene–haemin conjugates were initially investigated. Graphene was obtained by hydrazine reduction of exfoliated graphene oxide [9] prepared via Hummer’s method [39] . The immobilization of monomeric haemin on graphene via π–π stacking was conducted using our previously reported approach [37] . L -arginine oxidation reactions were conducted by dispersing the graphene–haemin catalyst in a pH 7.4 PBS buffer with 200 μM L -arginine, along with 5 mM H 2 O 2 as the oxidant ( Fig. 2a ). The L -arginine oxidation reaction could potentially result in multiple different products including NO or HNO. We have conducted extensive characterizations to demonstrate that the product is predominantly HNO. For product identification, the generated HNO dimerizes to form nitrous oxide over time, which is detectable by gas-phase Fourier transform infrared (FT-IR) spectroscopy [40] . The gas-phase FT-IR spectrum of the headspace gas of reaction vessel confirms the presence of nitrous oxide with two stretching bands at 2,211 and 2,235 cm −1 ( Supplementary Fig. 1 ). The NO stretching bands at 1,790 and 1,810 cm −1 are not observed, excluding NO as the product of the reaction. The headspace gas is also tested by gas chromatography–mass spectrometry (GC-MS) for nitrous oxide detection [41] , which further proves the existence of HNO ( Supplementary Fig. 2 ). In addition, chemiluminescence analysis, which can selectively detect p.p.b. levels of NO, but not HNO nor nitrous oxide, also demonstrates that there is no NO produced from the oxidation reaction ( Supplementary Fig. 3 ). The expected by-product L -citrulline is also tested by LC-MS [42] , further confirming the reaction pathway ( Supplementary Fig. 4 ). 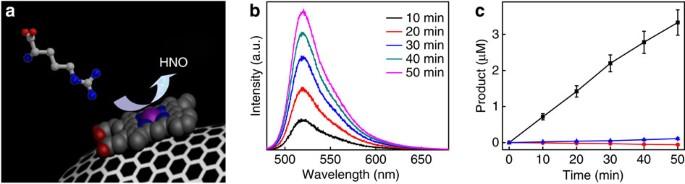Figure 2: Graphene–haemin conjugate-catalysed oxidation ofL-arginine. (a) A schematic illustration of graphene–haemin-catalysedL-arginine oxidation to produce HNO. (b) Relative fluorescence spectra at different reaction time obtained by DAF assay. (c) The HNO concentration determined by DAF assay. Black line represents product formation using graphene–haemin conjugate catalyst. Blue line represents product formation using free haemin catalyst. Red line represents product formation in a control experiment without catalyst. The size of the error bars represents the minimum to maximum values measured from at least three independent experiments. Figure 2: Graphene–haemin conjugate-catalysed oxidation of L -arginine. ( a ) A schematic illustration of graphene–haemin-catalysed L -arginine oxidation to produce HNO. ( b ) Relative fluorescence spectra at different reaction time obtained by DAF assay. ( c ) The HNO concentration determined by DAF assay. Black line represents product formation using graphene–haemin conjugate catalyst. Blue line represents product formation using free haemin catalyst. Red line represents product formation in a control experiment without catalyst. The size of the error bars represents the minimum to maximum values measured from at least three independent experiments. Full size image The above studies demonstrate that a graphene–haemin conjugate can function as an effective catalyst for the production of HNO. However, those methods are not capable of quantifying the generated HNO amount in reaction solution. Therefore, a fluorescence diaminofluorescein (DAF) assay was used. It has been documented that HNO can react with diaminofluorescein-2 to form diaminofluorescein-triazole with fluorescence emission [43] . The fluorescence spectrum was monitored at different time intervals ( Fig. 2b ), and the intensity increase of the emission peak at 515 nm was calibrated with the corresponding HNO concentrations ( Fig. 2c ). The DAF assay clearly shows the production of HNO immediately after the introduction of H 2 O 2 to a graphene–haemin-catalysed reaction mixture, while the control reaction without the graphene–haemin conjugate does not yield any signal ( Fig. 2c ). Significantly, for the reactions with the equivalent amount of haemin, the graphene–haemin catalysts exhibit a remarkably higher activity, while the free haemin hardly shows any catalytic activity at all ( Fig. 2c ). Such a difference in catalytic behaviour can probably be attributed to the monomeric molecular structure of haemin on graphene supports. For free haemin, the active catalytic sites are limited because of molecular aggregation of haemin to form inactive dimers. The catalytic turnover frequency of graphene–haemin is calculated to be 0.015 min −1 ( Fig. 2c ), which greatly exceeds that of the previously reported resin-supported system (0.0016, min −1 ) [36] . Moreover, graphene–haemin conjugates also exhibit exceptional catalytic activity stability, with nearly a constant turnover rate over a 50-min test period, while the previously reported resin-supported haemin could only catalyse the reaction for about 6 min before a total loss of its catalytic activity [36] . Graphene–haemin–GOx for HNO production Although, as demonstrated above, the graphene–haemin conjugates can effectively catalyse the oxidation of L -arginine to generate HNO, this reaction requires a relatively high concentration (~5 mM) of H 2 O 2 oxidant that is far above the physiological H 2 O 2 concentration (10 −9 ~10 −7 M) [44] . To apply the graphene–haemin catalyst for practical applications under physiological conditions, a mechanism to locally produce desired levels of H 2 O 2 is required. To this end, linking GOx to the graphene–haemin conjugates can offer an approach to elevate the local H 2 O 2 concentration through the oxidation of blood glucose. GOx was anchored via a N-hydroxysuccinimide–ethyl(dimethylaminopropyl) carbodiimide (NHS–EDC) coupling reaction and linked to the edge and defect site carboxyl groups of graphene. NHS–EDC coupling has been successfully used for the covalent linkage of GOx onto graphene oxide previously [45] . Stained transmission electron microscopy shows dark features of around 10 nm size distributed around the edges or defective sites of graphene, which is attributed to the successful linkage of GOx ( Supplementary Fig. 5 ). The formation of graphene–haemin–GOx is also supported by zeta potential measurements ( Supplementary Table 1 ). Once the graphene–haemin–GOx conjugates were obtained, H 2 O 2 production activity was tested in the presence of glucose and L -arginine ( Supplementary Fig. 6 ), demonstrating that GOx retains good activity after chemical linkage onto the graphene. The integrated catalysts were then used to catalyse the L -arginine oxidation reaction, and the HNO generation behaviour was studied using the DAF-based HNO assay. In pH 7.4 PBS buffer containing physiological concentrations of glucose (5 mM) and L -arginine (200 μM), the graphene–haemin–GOx conjugates produce HNO after a short activation stage (~5 min; Fig. 3a ). This lag might be due to the necessary accumulation of an adequate H 2 O 2 concentration at the surface of the graphene. For a series of control experiments, graphene–haemin–GOx catalysts in a solution of only glucose cannot produce any HNO, and a similar result was obtained for a solution containing only L -arginine, but not glucose ( Fig. 3a ). In a solution with both glucose and L -arginine, if only graphene–haemin conjugates or graphene–GOx conjugates alone are introduced, no HNO production is observed. Taken together, these findings clearly demonstrate that HNO production is observed only when the graphene–haemin–GOx conjugates, glucose and L -arginine are all present ( Fig. 3a ). The real-time reaction behaviour of this mixture was also monitored ( Fig. 3b ). Overall, the graphene–haemin–GOx conjugates can maintain good and stable activity over an extended period, and exhibits excellent recyclability ( Fig. 3b ). 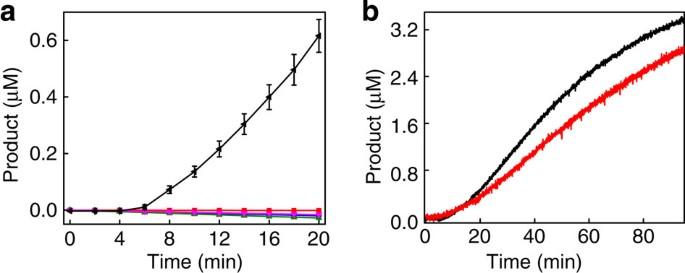Figure 3: HNO generation catalysed by graphene–haemin–GOx conjugates. (a) Graphene–haemin–GOx catalysed HNO generation and control experiments. The production of HNO was quantified using a DAF assay. Black line, graphene–haemin–GOx in glucose andL-arginine; red line, graphene–haemin in glucose andL-arginine; blue line, graphene–GOx in glucose andL-arginine; green line, graphene–haemin–GOx in glucose; pink line, graphene–haemin–GOx inL-arginine. The size of the error bars represents the minimum to maximum values measured from at least three independent experiments. (b) Real-time HNO production catalysed by graphene–haemin–GOx (black line) and by the recycled graphene–haemin–GOx catalysts (red line). Figure 3: HNO generation catalysed by graphene–haemin–GOx conjugates. ( a ) Graphene–haemin–GOx catalysed HNO generation and control experiments. The production of HNO was quantified using a DAF assay. Black line, graphene–haemin–GOx in glucose and L -arginine; red line, graphene–haemin in glucose and L -arginine; blue line, graphene–GOx in glucose and L -arginine; green line, graphene–haemin–GOx in glucose; pink line, graphene–haemin–GOx in L -arginine. The size of the error bars represents the minimum to maximum values measured from at least three independent experiments. ( b ) Real-time HNO production catalysed by graphene–haemin–GOx (black line) and by the recycled graphene–haemin–GOx catalysts (red line). Full size image Antithrombotic behaviour of graphene–haemin–GOx-embedded film Our studies have clearly demonstrated that graphene–haemin–GOx conjugates can function as effective catalysts for the generation of HNO with endogenous components. To further investigate whether the graphene–haemin–GOx conjugates can offer an effective solution for potential biomedical applications, we embedded the conjugates (at ~40 wt%) in a commercially available polyurethane (Tecophilic® SP-93A-100) that was then spin coated to form biocompatible films. Control thin film samples were also prepared with embedded graphene, graphene–haemin or graphene–GOx (at the same wt%). All the films were then immersed into platelet-rich rabbit blood plasma for 3 days, and then examined by scanning electron microscopy to evaluate the platelet adhesion characteristics [46] . Control films containing graphene, graphene–haemin or graphene–GOx exhibited very rough surfaces after blood contact, indicating obvious adhesion of a significant number of blood platelets ( Fig. 4a–c,e–g ). In contrast, the film containing graphene–haemin–GOx shows a minimum morphology change before and after blood contact ( Fig. 4d,h ), clearly demonstrating excellent antiplatelet function. 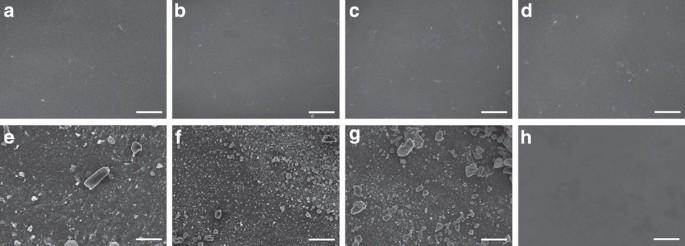Figure 4: Antithrombotic behaviour of biocompatible films containing graphene–haemin–GOx conjugates. Scanning electron microscopic (SEM) images of as-formed films containing (a) graphene, (b) graphene–haemin, (c) graphene–GOx and (d) graphene–haemin–GOx; and the respective films after immersing into platelet-rich rabbit blood plasma for 3 days: (e) graphene, (f) graphene–haemin, (g) graphene–GOx and (h) graphene–haemin–GOx. Only films containing graphene–haemin–GOx exhibit a minimum morphology change by SEM after immersion into blood plasma compared to control films of graphene, graphene–haemin or graphene–GOx. Scale bars, 10 μm. Figure 4: Antithrombotic behaviour of biocompatible films containing graphene–haemin–GOx conjugates. Scanning electron microscopic (SEM) images of as-formed films containing ( a ) graphene, ( b ) graphene–haemin, ( c ) graphene–GOx and ( d ) graphene–haemin–GOx; and the respective films after immersing into platelet-rich rabbit blood plasma for 3 days: ( e ) graphene, ( f ) graphene–haemin, ( g ) graphene–GOx and ( h ) graphene–haemin–GOx. Only films containing graphene–haemin–GOx exhibit a minimum morphology change by SEM after immersion into blood plasma compared to control films of graphene, graphene–haemin or graphene–GOx. Scale bars, 10 μm. Full size image By simultaneously conjugating haemin and GOx on graphene, we have created an integrated tandem catalyst that can drive a reaction cascade to allow for in situ generation of H 2 O 2 for the oxidation of L -arginine. This process can thus allow sustained generation of HNO from physiological glucose, L -arginine and blood oxygen. The embedment of such tandem catalysts into biocompatible films can create a surface coating with excellent antiplatelet characteristics, offering a potential solution to sustained generation of antithrombotic HNO species on medical devices when in contact with fresh blood. Overall, our studies demonstrate a general strategy to integrate molecular catalysts and enzymatic catalysts on the same platform for them to synergistically facilitate complex reaction pathways under mild physiological relevant conditions, and enable important chemical transformations not otherwise readily possible. It can have an impact on diverse areas including biomedicine and green chemistry. Preparation of graphene–haemin–GOx conjugates The preparation of graphene–haemin–GOx conjugates are followed stepwise via immobilization of haemin on graphene surface, and then linkage of GOx to the carboxyl groups at the edge and defect site of graphene. The graphene–haemin conjugates were prepared using the previously reported protocols [37] . Graphene–haemin conjugates were then mixed with NHS–EDC coupling agent for 2 h, centrifuged and washed, followed by stirring with 0.1 mg ml −1 GOx in pH 7.4 PBS buffer overnight for GOx linkage. Graphene–haemin–GOx conjugates were then centrifuged and washed with a pH 7.4 PBS buffer. Characterization of L -arginine oxidation reaction L -arginine oxidation reactions by graphene–haemin were carried out in the presence of 200 μM L -arginine and 5 mM H 2 O 2 in a pH 7.4 PBS buffer. L -arginine oxidation reactions by graphene–haemin–GOx were carried out in the presence of 200 μM L -arginine and 5 mM glucose in a pH 7.4 PBS buffer. The product was characterized using FT-IR, GC-MS, DAF assay and chemiluminescence. For FT-IR spectroscopy, the gas-phase FT-IR spectrum of the headspace gas was taken after 2-h reaction. For GC-MS measurement, the headspace gas was injected into an Agilent 6890-5975 GC-MS with a 30 m Rt®-Q-Bound column (Resteck Co, Columbia, MD) at an operating oven temperature of 45 °C under 14.6 p.s.i. helium carrier gas. For the DAF assay, 10 μM DAF-2 was added to the reaction solution. The excitation wavelength was 448 nm. At each time interval, florescence spectra were obtained from an average of five accumulations. Peak intensities of 515 nm were also monitored continuously for reaction catalysed by graphene–haemin–GOx conjugates. For chemiluminescence, the solution after 2-h reaction was bubbled with Ar and the products were measured via a chemiluminescence NO Analyzer TM , Model 280 (Sievers Instruments, Boulder, CO). In situ measurements were also carried out. Antithrombotic film fabrication and antithrombotic studies Tecophilic® SP-93A-100 polyurethane was dissolved in tetrahydrofuran to make a solution of 40 mg ml −1 . Graphene, graphene–haemin, graphene–GOx or graphene–haemin–GOx were then mixed with polymer solution and films cast on silicon substrates by spin coating. Films were peeled off after drying. Arterial blood from New Zealand white rabbits, weighing 2.5–3 kg, was drawn into a 9:1 volume of a blood:anticoagulant citrate solution. The National Institutes of Health guidelines for the care and use of laboratory animals (NIH Publication number 85–23 Rev. 1985) were observed throughout. The citrated whole blood was centrifuged at 110 g for 15 min at 22 °C. Platelet-rich plasma was collected from the supernatant. Films were first immersed in a pH 7.4 PBS buffer containing 200 μM L -arginine and 5 mM glucose for 30 min, and then immersed in platelet-rich plasma for 3 days. Films were then washed with pH 7.4 PBS buffer, dried and sputtered with gold for platelet aggregation and thrombus formation investigation by JEOL JSM-6700F FE-SEM. How to cite this article: Xue, T. et al. Integration of molecular and enzymatic catalysts on graphene for biomimetic generation of antithrombotic species. Nat. Commun. 5:3200 doi: 10.1038/ncomms4200 (2014).